Model studies of force-dependent kinetics of multi-barrier reactions According to transition state theory, the rate of a reaction that traverses multiple energy barriers is determined by the least stable (rate-determining) transition state. The preceding (‘inner’) energy barriers are kinetically ‘invisible’ but mechanistically significant. Here we show experimentally and computationally that the reduction rate of organic disulphides by phosphines in water, which in the absence of force proceeds by an equilibrium formation of a thiophosphonium intermediate, measured as a function of force applied on the disulphide moiety yields a usefully accurate estimate of the height of the inner barrier. We apply varying stretching force to the disulphide by incorporating it into a series of increasingly strained macrocycles. This force accelerates the reduction, even though the strain-free rate-determining step is orthogonal to the pulling direction. The observed rate–force correlation is consistent with the simplest model of force-dependent kinetics of a multi-barrier reaction. Extensive empirical evidence indicates that kinetic stabilities of diverse reactive sites within a polymer are affected when the polymer is stretched by application of tensile force. Such force-dependent reactivity is thought to account for the behaviour of polymeric materials, melts and solutions under load, may be exploited to yield new stress-responsive, actuating and energy transducing materials [1] , [2] , [3] , [4] , [5] , [6] , [7] , [8] , [9] , [10] and may even allow characterization of transition states. [11] Considerable theoretical, [3] , [12] , [13] , [14] , [15] , [16] , [17] , [18] , [19] computational [13] , [20] , [21] , [22] , [23] , [24] , [25] , [26] and experimental [27] , [28] , [29] , [30] , [31] , [32] , [33] , [34] effort has been devoted to refine and validate a model of force-dependent kinetics for elementary (single-barrier) reactions. Yet many reactions proceed through one or more intermediates, that is, multiple activation barriers separate the reactant(s) from the product(s). Examples include solvolysis of esters and amides (the A AC 2 and B AC 2 mechanisms), nucleophilic displacements (D and A mechanisms), additions, eliminations, cycloreversions, retro-Diels-Alder and redox reactions. [35] , [36] Little experimental or theoretical work has been reported on how stretching force affects the kinetics and mechanisms of multi-barrier reactions. Non-linear correlations between stretching force and the apparent activation energy of unfolding of several biopolymers was interpreted as indicating force-induced shift of the rate-determining step to an inner barrier (that is, a barrier that in the absence of force precedes the rate-determining step), but alternative explanations were proposed as well. [37] , [38] , [39] , [40] , [41] , [42] , [43] , [44] A major theoretical challenge of extending the current models of force-dependent kinetics to multi-barrier reactions is the likelihood that stretching force affects individual steps of such reactions very differently because molecular dimensions change non-monotonically along the reaction paths. A stretched polymer in single-molecule force or elongational flow experiments can be thought of as a molecule coupled, at two of its atoms, to a constraining potential that exerts a stretching force on these two atoms. [3] , [5] , [13] , [18] , [45] , [46] An activation barrier for a reaction in such a polymer will depend on stretching force if the strain energy of the constraining potential is different at the top and the bottom of the barrier (that is, at the transition state and reactant or intermediate). To a good approximation, this strain energy change between two points on the energy surface (also known as work potential) is proportional to the difference of the separation of the two atoms at which the potential acts (so called pulling axis) at these points. For example, if the separation of the constrained atoms remains the same in a transition state and the corresponding reactant or the intermediate (that is, the pulling axis is orthogonal to the reaction coordinate), a stretching force will not affect the kinetics of that step. Even during multi-barrier molecular dissociations, certain internuclear distances that increase to infinity in the products may not change or even contract over some elementary steps. 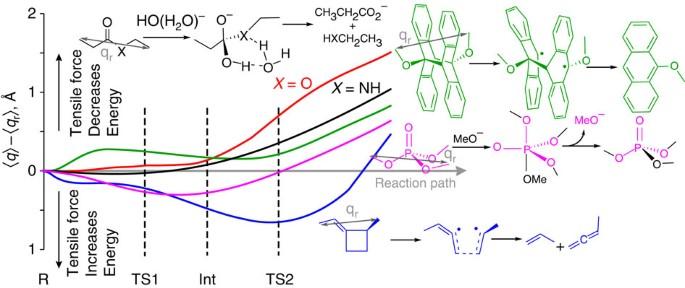Figure 1: Non-monotonous change of terminal distances along the reaction paths. The reaction schemes show the reactant, the intermediate and the product and the plotted distance (grey arrows)1,3,7,8. The computational details are described in the Methods;signifies Boltzmann averaging over multiple conformers comprising the stationary states; for degenerate exchange of CH3O−in O=P(OCH3)3, the separation between the leaving group and each spectator CH3group was included in calculatingq. Figure 1 illustrates the diversity of patterns of changes in the terminal C … C distance along the steepest-descent paths of several double-barrier dissociation reactions of potential importance in the development of stress-responsive polymers. Figure 1: Non-monotonous change of terminal distances along the reaction paths. The reaction schemes show the reactant, the intermediate and the product and the plotted distance (grey arrows) [1] , [3] , [7] , [8] . The computational details are described in the Methods; signifies Boltzmann averaging over multiple conformers comprising the stationary states; for degenerate exchange of CH 3 O − in O=P(OCH 3 ) 3 , the separation between the leaving group and each spectator CH 3 group was included in calculating q . Full size image Hydrolysis of esters and amides (red and black lines, Fig. 1 ) represents the simplest case of force-dependent kinetics of multi-barrier dissociations: the first of the two barriers is both rate determining and orthogonal to the pulling axis (that is, not accompanied by changes in the terminal C … C separation). Consequently, the dissociation rate is expected to be force-independent, in agreement with reported computational and experimental data. [47] , [48] In comparison, tensile force probably inhibits dissociation of methylethylidene cyclobutane (blue, Fig. 1 ). A very interesting situation arises if the second barrier is rate determining in the absence of strain. Such reactions may manifest force-dependent kinetics even if this second step is orthogonal to the pulling axis and the first (or ‘inner’) barrier may become rate-determining above a threshold force as illustrated in Fig. 2 . 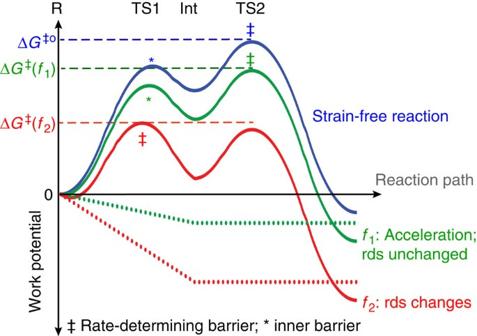Figure 2: The simplest model of a double-barrier reaction in the presence of force. The example has the second step orthogonal to the pulling axis. The inner barrier (*) in the absence of force (blue curve) becomes rate determining (‡) when sufficient force is imposed across a suitable pair of the atoms of the reactant (red curve). Because the second step is orthogonal to the pulling axis (that is, the constrained distance does not change between the intermediate and second transition state), the rate-determining step changes at applied forcef2because the force stabilizes the intermediate more than the first transition state. Consequently, the intermediate has to scale a larger barrier to revert to the reactants than to yield the product. Smaller forcef1does not change the reaction mechanism but still accelerates the reaction by suppressing reversion of the intermediate to the reactant. The reaction energy profiles atf1andf2(green and red lines) are obtained by adding the change in the strain energy of the constraining potential (‘work potential’, dotted lines) to the reaction profile in the absence of force (blue line). Figure 2: The simplest model of a double-barrier reaction in the presence of force. The example has the second step orthogonal to the pulling axis. The inner barrier (*) in the absence of force (blue curve) becomes rate determining (‡) when sufficient force is imposed across a suitable pair of the atoms of the reactant (red curve). Because the second step is orthogonal to the pulling axis (that is, the constrained distance does not change between the intermediate and second transition state), the rate-determining step changes at applied force f 2 because the force stabilizes the intermediate more than the first transition state. Consequently, the intermediate has to scale a larger barrier to revert to the reactants than to yield the product. Smaller force f 1 does not change the reaction mechanism but still accelerates the reaction by suppressing reversion of the intermediate to the reactant. The reaction energy profiles at f 1 and f 2 (green and red lines) are obtained by adding the change in the strain energy of the constraining potential (‘work potential’, dotted lines) to the reaction profile in the absence of force (blue line). Full size image Here we report an atomistically tractable model reaction to test these predictions. We demonstrate that the shape of the experimental force–rate correlation is characteristic of a shift of the rate-determining step to the ‘inner’ barrier above a threshold force and the force–rate correlation above this force yields usefully accurate estimate of the strain-free rate constant for the formation of the intermediate. The latter is important because for most reactions that proceed by an equilibrium formation of a reaction intermediate, the parameters of this ‘inner’ barrier cannot be extracted from bulk kinetic measurements. Strategy As highlighted recently, [5] the relationship between the kinetic stability of a reactive moiety and the restoring force of its molecular coordinates is often independent of whether the moiety is part of a stretched polymer or a suitably designed strained macrocycle. This independence enables predictions of chemically driven micromechanical behaviour of polymers and experimental tests of models of such behaviour using simple non-polymeric substrates. [32] Here we used this approach to study force-dependent kinetics of reduction of aliphatic disulphides, RSSR, by phosphines, PR 3 ′, in aqueous medium. The strain-free mechanism is shown in Fig. 3a ; [49] , [50] , [51] , [52] in neutral solution, the reduction of unstrained disulphides proceeds by rate-determining hydrolysis of a thiophosphonium intermediate. Because reversion of this intermediate to the disulphide requires a thiolate nucleophile, which can be (partially) protonated by acid, reduction of disulphides by phosphines is one of the few reactions in which the rate constant for the formation of a highly unstable reaction intermediate can be measured. By comparing this rate constant derived from the pH-dependence of the reduction rate of an unstrained disulphide with the one derived from the rate versus force correlations for a series of strained disulphides using the model in Fig. 2 , the model can be tested experimentally. 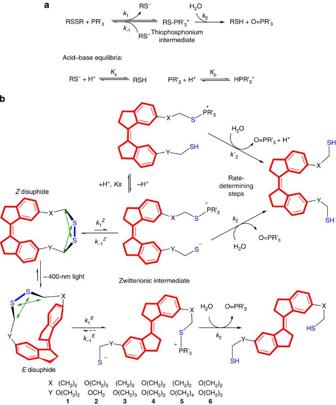Figure 3: The mechanism of reduction of disulphides by a phospine in H2O. (a) Acyclic disulphides. (b) A series of strain-free (Z) and increasingly strained (E) cyclic disulphides used to study the effect of stretching force on the kinetics and mechanism of a pre-equilibrium reaction. The strain of the disulphide moiety in the macrocycles was quantified as the restoring force of the two H2C…S local coordinates (green arrows). Restoring force that develops in an elastically deformed object, opposes further deformation and is responsible for the recovery of the original shape after load removal. In the harmonic approximation, the molecular compliance matrix relates the restoring force of a local coordinate of a molecule both to the absolute distortion of this coordinate and to the externally imposed force. The restoring force is rigorously defined both at the continuum and atomistic levels,3connecting the two descriptions of the response of an object to load. It is particularly valuable in describing the reaction kinetics of stretched polymers, where partial relaxation of non-reactive molecular degrees of freedom far removed from the reactive site makes large contributions to activation barriers. The restoring force provides a simple estimate of this contribution without treating such molecular coordinates explicitly. Figure 3: The mechanism of reduction of disulphides by a phospine in H 2 O. ( a ) Acyclic disulphides. ( b ) A series of strain-free ( Z ) and increasingly strained ( E ) cyclic disulphides used to study the effect of stretching force on the kinetics and mechanism of a pre-equilibrium reaction. The strain of the disulphide moiety in the macrocycles was quantified as the restoring force of the two H 2 C … S local coordinates (green arrows). Restoring force that develops in an elastically deformed object, opposes further deformation and is responsible for the recovery of the original shape after load removal. In the harmonic approximation, the molecular compliance matrix relates the restoring force of a local coordinate of a molecule both to the absolute distortion of this coordinate and to the externally imposed force. The restoring force is rigorously defined both at the continuum and atomistic levels, [3] connecting the two descriptions of the response of an object to load. It is particularly valuable in describing the reaction kinetics of stretched polymers, where partial relaxation of non-reactive molecular degrees of freedom far removed from the reactive site makes large contributions to activation barriers. The restoring force provides a simple estimate of this contribution without treating such molecular coordinates explicitly. Full size image We mimicked the strain that would be imposed on the disulphide moiety in a stretched polymer using a series of increasingly strained macrocyclic disulphides, E 1 – E 6 ( Fig. 3b ). We previously demonstrated that when the strain of a reactive moiety in such macrocycles is quantified as a restoring force of a properly chosen local molecular coordinate, the rate–force correlations measured with a series of macrocycles and in polymers stretched in single-molecule force experiments are equivalent. [32] Importantly, although the first step of reduction (formation of the thiophosphonium zwitterion) is coupled to changes in the molecular geometry of the stiff stilbene moiety (red, Fig. 3b ), the second (hydrolysis) step is not. In other words, the pulling axis is orthogonal to the rate-determining elementary step in the absence of force. This orthogonality is maintained even if the reaction occurs in a polymer stretched externally. We resorted to studying a non-polymeric disulphide because mechanistic and computational studies required to test models of force-dependent reactivity cannot yet be performed on polymers. Synthesis and kinetic measurements We synthesized strain-free Z disulphides ( Fig. 3b ), which served as reference for analysis of the reduction kinetics of the strained E analogues (see below), following the scheme in Fig. 4 .We measured the kinetics of reduction of these strain-free disulphides with large excess of triphenylphosphine (PPh 3 ) or methyldiphenylphosphine (PPh 2 CH 3 ) in H 2 O:CH 3 CN (3:1 mol) at 60 o C under rigorously anaerobic conditions. The compositions of all reaction mixtures were monitored for at least three half-lives by reverse-phase HPLC with aqueous CH 3 CN as eluent using an inert internal standard (see Supplementary Tables S3 and S4 for retention times and separation conditions). At μM concentrations of the cyclic disulphide, the reactions were first order in both phosphine and disulphide and yielded dithiol and phosphine oxides as the sole products, as confirmed independently by 1 H-NMR and HRMS measurements. No reaction was observed in the absence of H 2 O and no intermediate could be detected either in aqueous or anhydrous CH 3 CN, which is consistent with density functional theory (DFT) calculations of the free energy of formation of the zwitterionic intermediate in Z 1 – Z 6 being >8 kcal mol −1 . 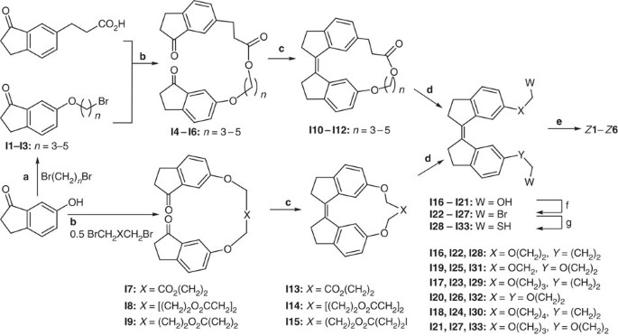Figure 4: Synthesis of macrocyclic disulphidesZ1–Z6. Summary of synthetic conditions: (a) Bu4NBr, K2CO3, acetone, reflux; (b) Bu4NBr, K2CO3, DMF, 65 °C; (c) TiCl4, Zn, THF, reflux; (d) LiAlH4, THF, reflux; (e) I2, NEt3, CHCl3, 25 °C; (f) CBr4, PPh3, acetone, CH2Cl2, 25°C; (g) thiourea, DMF, 80 °C, then NaOH, 25 °C, then HCl, 25 °C. See the Methods section for the synthetic protocols andSupplementary Tables S1 and S2for the spectroscopic characterization and reaction yields. Figure 4: Synthesis of macrocyclic disulphides Z 1– Z 6. Summary of synthetic conditions: ( a ) Bu 4 NBr, K 2 CO 3 , acetone, reflux; ( b ) Bu 4 NBr, K 2 CO 3 , DMF, 65 °C; ( c ) TiCl 4 , Zn, THF, reflux; ( d ) LiAlH 4 , THF, reflux; ( e ) I 2 , NEt 3 , CHCl 3 , 25 °C; ( f ) CBr 4 , PPh 3 , acetone, CH 2 Cl 2 , 25 ° C; ( g ) thiourea, DMF, 80 °C, then NaOH, 25 °C, then HCl, 25 °C. See the Methods section for the synthetic protocols and Supplementary Tables S1 and S2 for the spectroscopic characterization and reaction yields. Full size image The differential rate law for reduction of disulphides 1 – 6 is given by equations (1 and 2). To estimate the rate constants for the formation of the strain-free zwitterionic intermediates ( Fig. 3b ), we measured the reduction kinetics of disulphides Z 1 – Z 6 in the presence of triflic acid (100 μM–3 mM). As predicted by equation (2), the reduction accelerates with H + concentration ( Supplementary Tables S5 and S6 ). Least-square fitting of measured bimolecular rate constants, k Z , to equation (2) yielded rate constants for the formation of the zwitterionic intermediate, k 1 Z ( Table 1 ). These values are similar to those reported for reduction of simple alkyl disulfides by phenyl phosphines under strong basic conditions, where the formation of the RS-PR 3 ′ + intermediate is thought to be rate limiting. [51] Consistent with the mechanism in Fig. 3b , ( k 1 Z / k Z − 1) −1 versus [H + ] correlations were linear ( Fig. 5 ). The variation of k 1 Z values across disulphides Z 1 – Z 6 probably reflects the electronic influence of the linkers connecting the disulphide moiety to stiff stilbene (red, Fig. 3b ). Table 1 Measured reduction kinetics of disulphides 1–6. 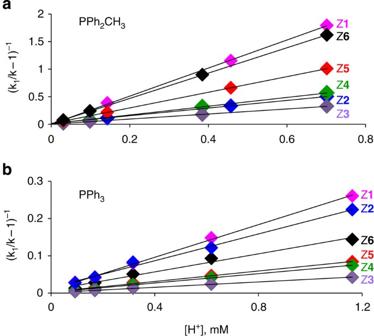Figure 5: Acceleration of the reduction of strain-free disulphidesZ1–Z6 in acidic solution. Linearity of (k1Z/kZ−1)−1versus [H+] graphs (a: by PPh2Me;b: by PPh3) is consistent with reduction of disulphidesZ1–Z6proceeding by the mechanism inFig. 3b. Lines are linear least-squares fits. The intercepts (k2/k−1) range from (1.7±0.2) × 10−2to (1.1±0.5) × 10−3, indicating that under neutral conditions, a strain-free zwitterionic intermediate is 60 to 103times more likely to revert back to the disulphide than to undergo hydrolysis to the products, again consistent with the postulated reaction mechanism. The intercept-to-slope ratios (Ksk2′/k2) averaged ~3 μM for reduction with PPh2CH3and ~40 μM for reduction with PPh3and equal proton concentration, [H+], at which half of the reaction proceeds through the protonated intermediate. The listed values are averages of three independent measurements; s.d. are smaller than the size of the markers. The plotted data is tabulated inSupplementary Tables S5–S7. Full size table Figure 5: Acceleration of the reduction of strain-free disulphides Z 1– Z 6 in acidic solution. Linearity of ( k 1 Z / k Z −1) −1 versus [H + ] graphs ( a : by PPh 2 Me; b : by PPh 3 ) is consistent with reduction of disulphides Z 1 – Z 6 proceeding by the mechanism in Fig. 3b . Lines are linear least-squares fits. The intercepts ( k 2 / k −1 ) range from (1.7±0.2) × 10 −2 to (1.1±0.5) × 10 −3 , indicating that under neutral conditions, a strain-free zwitterionic intermediate is 60 to 10 3 times more likely to revert back to the disulphide than to undergo hydrolysis to the products, again consistent with the postulated reaction mechanism. The intercept-to-slope ratios ( K s k 2 ′/ k 2 ) averaged ~3 μM for reduction with PPh 2 CH 3 and ~40 μM for reduction with PPh 3 and equal proton concentration, [H + ], at which half of the reaction proceeds through the protonated intermediate. The listed values are averages of three independent measurements; s.d. are smaller than the size of the markers. The plotted data is tabulated in Supplementary Tables S5–S7 . Full size image To study force-dependent kinetics of disulphide reduction by phosphines without the complications inherent to polymers and micromanipulation techniques we used the E isomers of disulphides 1 – 6 ( Fig. 3b ). The molecular strap containing the disulphide moiety, which bridges the two phenyl rings of stiff stilbene is too short to accommodate the strain-free E geometry of the central C=C bond. Consequently, photoisomerization of Z stiff stilbene in Z 1 – Z 6 creates strained analogues in which the distribution of kinetically significant molecular strain within the reactive moiety approximates that of the same moiety in a stretched oligomer. [3] Photostationary states containing up to 50% of strained disulphides E 1 – E 6 were obtained by irradiation of ~20 μM solutions of the Z analogues in CH 3 CN under rigorously anhydrous and anaerobic conditions ( Supplementary Table S2 ). Most kinetic measurements were conducted on these photostationary states to minimize the measurement error of the ratio of the rate constants, k E / k Z (see below). Other conditions were identical to those used for Z 1 – Z 6 . Table 1 lists the measured rate constants in the absence of added [H + ]. Unlike the reduction of the Z disulphides, triflic acid did not affect the apparent bimolecular rate constants for the reduction of the E analogues ( Supplementary Table S8 ). DFT calculations To use the measured data to test the model of the kinetics of double-barrier reaction under stretching force ( Fig. 2 ) we first optimized all thermally accessible conformers of both isomers of disulphides 1 – 6 as well as the transition states for the formation of the zwitterionic intermediates ( Fig. 3b ) at the B3LYP/6-311+G(d) level of the DFT with H 2 O-parameterized SMD model [53] as a continuum representation of the reaction solvent ( Supplementary Tables S9 and S10 list the key parameters of the reactant and transition states and Supplementary Tables S11–S13 list the parameters of individual conformers). These calculations yielded free energies of activation of the first step in a good agreement with the measured ( E isomers) or fitted ( Z isomers) values ( Table 2 : the mean absolute deviation of 1.3 kcal mol −1 ). Table 2 Activation free energies of disulphide reduction. Full size table We quantified the strain of the disulphide moiety in each macrocycle as the ensemble-average restoring force of the non-bonding H 2 C … S distances (green arrows, Fig. 3b ), which we previously showed to be a useful 1-dimensional representation of the full reaction coordinate of S N 2 displacement at S. [29] We obtained the restoring forces by comparing the ensemble-average H 2 C … S distances in each macrocycle against the calibration curve relating the equivalent ensemble-average distances and their restoring forces in Et 2 S 2 with an external stretching force applied across the terminal C atoms ( Fig. 6 ), obtained computationally as described in the Methods section. 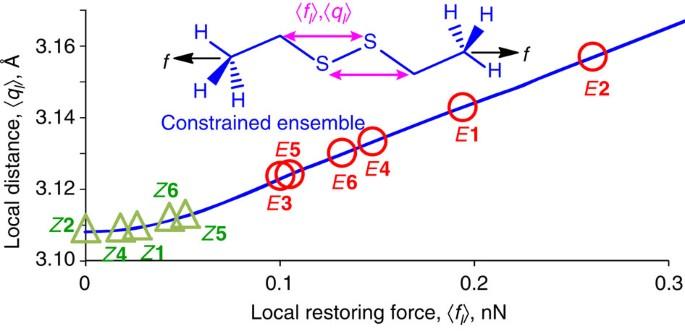Figure 6: The calculated distance–force correlation of the H2C…S coordinate of aliphatic disulphide. The restoring forces of the disulphide moieties in1–6,fl, were obtained by comparing computed H2C…S separations,ql, in disulphides1–6(green arrows inFig. 3b) to the force-extension curve for the ensemble of Et2S2with the stretching force applied across the terminal C atoms. All calculations were at the B3LYP/6-311+G(d) level in SMD. InZ3ql=3.106 Å, corresponding to a compressive force of 35 pN and is not shown on the graph. The plotted data is tabulated inSupplementary Tables S9 and S14. [25] , [32] Figure 6: The calculated distance–force correlation of the H 2 C … S coordinate of aliphatic disulphide. The restoring forces of the disulphide moieties in 1 – 6 , f l , were obtained by comparing computed H 2 C … S separations, q l , in disulphides 1 – 6 (green arrows in Fig. 3b ) to the force-extension curve for the ensemble of Et 2 S 2 with the stretching force applied across the terminal C atoms. All calculations were at the B3LYP/6-311+G(d) level in SMD. In Z 3 q l =3.106 Å, corresponding to a compressive force of 35 pN and is not shown on the graph. The plotted data is tabulated in Supplementary Tables S9 and S14 . Full size image The measured reduction rate constant of an E disulphide, k E , normalized to the extrapolated rate constant for the formation of the zwitterionic intermediate in the corresponding Z analogue ( k 1 Z ), ln (k E / k 1 Z ) are plotted in Fig. 7a against the restoring force of the local coordinate (green arrows, Fig. 3b ), in the E reactant, f l E . We analyse the ln (k E / k 1 Z ) ratio to eliminate rate variations due to the distinct stereoelectronic contributions of different linkers across the series of macrocycles. In our method, different linkers are necessary to control the force exerted on the reactive site, but they may introduce rate variability among different macrocycles that is unrelated to strain. When force on a reactive site can be varied without changing the chemical composition in its vicinity (for example, in single-molecule force experiments on polymers), such normalization of rate constants becomes unnecessary. 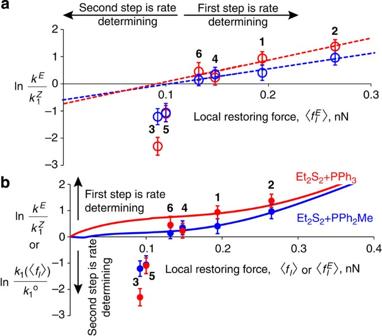Figure 7: Reduction kinetics as a function of the force applied to the disulphide moiety. (a). Log of the ratio of the reduction rate constants of strained disulphidesE1–E6to the rate constants of the formation of the zwiterionic intermediate in strain-freeZ1–Z6analogues with PPh3(red) and PPh2CH3(blue) versus the ensemble-average restoring force of the H2C…S coordinate of the disulphide moiety (green arrows,Fig. 3b) inE1–E6,flE. Broken lines are linear least-squares fits to data for disulphides1,2,4, and6. (b) The calculated acceleration of the first step of disulphide reduction (formation of the thiophosphonium intermediate, solid lines) and measured acceleration of reduction of disulphides1–6(points) versus local restoring force. As described elsewhere in the manuscript, the deviation of the measured ln(kE/k1Z) ratio for disulphides3and5from the computed ln(k1(fl)/k1o) values (solid lines) is consistent with the stretching force applied to the disulphide moiety inE3andE5being too small to shift the rate-determining step to the formation of the zwitterionic intermediate (that is, similar to the green line inFig. 2). The error bars reflect the standard deviations of three independent measurements. The nonlinearity of ΔΔG1‡ln(k1(fl)/k1o) versusfcorrelations (solid lines) results primarily from the strong dependence of the difference in the constrained distance between the reactant and the transition state (Supplementary Figs S1 and S2). The plotted data are tabulated inTable 1andSupplementary Table S14. The ΔG1‡(fl) correlations up to 1.5 nN are shown inSupplementary Fig. S3. Figure 7: Reduction kinetics as a function of the force applied to the disulphide moiety. ( a ). Log of the ratio of the reduction rate constants of strained disulphides E 1 – E 6 to the rate constants of the formation of the zwiterionic intermediate in strain-free Z 1 – Z 6 analogues with PPh 3 (red) and PPh 2 CH 3 (blue) versus the ensemble-average restoring force of the H 2 C … S coordinate of the disulphide moiety (green arrows, Fig. 3b ) in E 1 – E 6 , f l E . Broken lines are linear least-squares fits to data for disulphides 1 , 2 , 4 , and 6 . ( b ) The calculated acceleration of the first step of disulphide reduction (formation of the thiophosphonium intermediate, solid lines) and measured acceleration of reduction of disulphides 1 – 6 (points) versus local restoring force. As described elsewhere in the manuscript, the deviation of the measured ln (k E / k 1 Z ) ratio for disulphides 3 and 5 from the computed ln (k 1 ( f l )/ k 1 o ) values (solid lines) is consistent with the stretching force applied to the disulphide moiety in E 3 and E 5 being too small to shift the rate-determining step to the formation of the zwitterionic intermediate (that is, similar to the green line in Fig. 2 ). The error bars reflect the standard deviations of three independent measurements. The nonlinearity of ΔΔ G 1 ‡ ln( k 1 ( f l )/ k 1 o ) versus f correlations (solid lines) results primarily from the strong dependence of the difference in the constrained distance between the reactant and the transition state ( Supplementary Figs S1 and S2 ). The plotted data are tabulated in Table 1 and Supplementary Table S14 . The Δ G 1 ‡ ( f l ) correlations up to 1.5 nN are shown in Supplementary Fig. S3 . Full size image The two distinct kinetic regimes (at f l E below and above ~120 pN) apparent across the series of the disulphides ( Fig. 7a ) are consistent with the simple picture in Fig. 2 . At low forces of weakly strained disulphides E 3 and E 5 the reduction is accelerated without a change in the rate-determining step ( cf. green trace, Fig. 2 ), as evidenced by the observation that the apparent rate constants of reduction of E 3 and E 5 exceeds that of their strain-free analogues, Z 3 and Z 5 , but remains smaller than that of the first reduction step, that is, the formation of the strain-free zwitterionic intermediate (that is, k Z < k E < k 1 Z , for example, 0.19±0.04, 1.91±0.19 and 5.5±0.6 M −1 s −1 , respectively, for 5 ). At higher forces (disulphides E 1 , E 2 , E 4 , and E 6 ), the apparent reduction rate constants k E , both exceed those of the formation of the zwitterionic intermediate of the corresponding strain-free Z analogues, and are independent of the solution acidity ( Supplementary Table S8 ), suggesting the shift of the rate-determining step to the previously inner barrier ( cf . red line, Fig. 2 ). Indeed, the slopes of the linear regression of the vs. f l E data above 120 pN (broken lines in Fig. 7a ), normalized to thermal energy (0.25 and 0.35 Å for the reduction by PPh 2 CH 3 and PPh 3 , respectively) are reasonably close to the average elongation of the H 2 C … S separation from the reactant to the transition state in macrocyclic disulphides (0.16 and 0.24 Å, Supplementary Tables S9 and S10 ; Supplementary Figs. S1 and S2 ), in accord with the simplest model of single-barrier force-dependent kinetics. [54] To confirm the conclusion that reduction of disulphides E 1 , E 2 , E 4 , and E 6 is limited by the force-dependent kinetics of the formation of the zwitterionic intermediate, rather than the force-independent hydrolysis of the zwitterionic intermediate, as in the strain-free disulphide, we calculated (at the B3LYP/6-311+G (d) level in H 2 O-parameterized SMD [53] ) the activation free energy of the first step in reduction of Et 2 S 2 by PPh 3 and PPh 2 CH 3 ( Fig. 3a ) as a function of the stretching force applied across the terminal C atoms of Et 2 S 2 , using previously described methodology. [25] , [32] Stretching force lowers the first barrier for both phosphines as indicated by positive values of ln[ k 1 ( f )/ k 1 o ], where k 1 o is the rate constant in the absence of force. The measured values of for disulphides 1 , 2 , 4 , 6 follow this trend closely, suggesting that the acceleration of reduction of E 1 , E 2 , E 4 and E 6 relative to their strain-free Z analogues can be attributed to force-dependent lowering of the first (now rate-determining) barrier. The deviation of the measured ln (k E / k 1 Z ) ratio for disulphides 3 and 5 from the computed ln (k 1 ( f l )/ k 1 o ) correlation is consistent with the rate-determining step in these weakly strained disulphides being the same as in the absence of strain, that is, hydrolysis of the zwitterionic intermediate ( Fig. 3b ). We conclude that, at least for the reduction of a disulphide by a phosphine, the simple model of force-dependent kinetics of a multi-barrier reaction shown in Fig. 2 is valid. Although the second step, which is rate-determining at low-stretching forces, is orthogonal to the pulling axis and is therefore not affected by force, the overall reaction is accelerated by force because force suppresses reversion of the intermediate to the reactant. The force–rate correlation shows two kinetic regimes and a usefully accurate estimate of the rate constant for the formation of strain-free intermediate is obtained from extrapolating the high-force regime to zero force. The accuracy of the extrapolated strain-free ‘inner’ barrier height (or the corresponding rate constant) depends strongly on identifying the minimum force corresponding to the change in the rate-determining step and is thus facilitated by the fairly sharp delineation of the two kinetic regimes in Fig. 7a . The existence of multiple energy barriers preceding the rate-determining transition states may obscure such turnover regimes, potentially complicating the molecular interpretation of rate–force correlations. Distinct kinetic regimes at small and large forces are sometimes observed in single-molecule force experiments [43] but whether they represent changes in the rate-determining step remains uncertain. [45] , [55] Applying the methodology described above to other reactions that traverse multiple barriers (for example, those in Fig. 1 ) would help define the limits of applicability of the simple picture in Fig. 2 . General Structures of synthetic intermediates I3 – I33 are shown in Figure 4 ; the reaction yields and spectroscopic characterization are in Supplementary Tables S1 and S2 . The disulphides 1 – 6 and the diols I28 – I33 were first reported in Kucharski et al . [29] Commercial reagents of the highest available purity from Aldrich or Fisher were used without further purification unless stated otherwise. Water was obtained from a Milli-Q water purification system. Analytical and preparative thin-layer chromatography was performed on silica gel 60 from Fisher and Aldrich. The concentrations of aqueous trifluoromethanesulphonic acid (TfOH) solutions were determined by titration with commercial standards. Irradiation was performed in vessels sealed under N 2 using high-intensity diode light sources from Opto Technology with light output at 375±7 nm. Light intensity was controlled with a custom-made constant-current controller. UV–vis absorption spectra were recorded on a Cary 50 UV–vis spectrophotometer. The diode light source was oriented 90° from the spectrophotometer beam path so that UV–vis absorbance spectra could be measured during irradiation to monitor reaction progress. Analytical HPLC was performed on a Shimadzu Prominence LC system with LC-20AT solvent delivery unit, DGU-20A5 degasser, SPD-M20A photodiode array detector, CBM-20A system controller and Rheodyne 7725i manual injector, with either a J. T. Baker C18 column (25 cm × 4.6 mm, 5 μm particles), Supelco C18 column (15 cm × 4.6 mm, 5 μm particles), or Agilent Hypersil AA-ODS (C18) column (20 cm × 2.1 mm, 5 μm particles). High-resolution mass spectrometry (HRMS) was performed on a Micromass 70-VSE mass spectrometer (EI) or a Waters Q-Tof Ultima mass spectrometer (ESI) at the University of Illinois Mass Spectrometry Center. NMR spectra of macrocycles 1–6 and synthetic intermediates were recorded on 400 Unity-INOVA Varian spectrometers at room temperature (~20 °C). Chemical shifts are reported in p.p.m. downfield from that of tetramethylsilane and are referenced to the residual 1 H resonances of the deuterated solvents. 31 P{1H} resonances are reported in p.p.m. downfield from 85% H 3 PO 4 , but were not externally referenced. Synthesis of I1–I3 6-Hydroxyindanone (0.3 g), K 2 CO 3 (1.5 eq. ), N( n -C 4 H 9 ) 4 Br (0.1 eq.) and Br(CH 2 ) n Br ( n =3, 4 or 5 for I1 , I2 or I3 , respectively, 6.0 eq.) in acetone (20 ml) were refluxed for ~16 h, cooled to room temperature (RT), and poured in H 2 O (60 ml). The product was extracted with CH 2 Cl 2 (3 × 40 ml). The organic fractions were dried over MgSO 4 , filtered and concentrated under reduced pressure. The crude product was purified by flash chromatography with hexanes followed by CH 2 Cl 2 to afford I1 – I3 as pale yellow solids. Synthesis of I4–I6 3-(6-Indan-1-one)propionic acid (0.3 g), K 2 CO 3 (1.5 eq. ), I1 , I2 or I3 (1.0 eq. ), and N( n -C 4 H 9 ) 4 Br (0.1 eq.) in dry DMF (20 ml) were heated at 65 °C for ~20 h. The mixture was cooled to RT, diluted with CH 2 Cl 2 (100 ml) and washed with brine (4 × 100 ml). The organic fractions were dried over MgSO 4 , filtered and concentrated under vacuum to afford I4 – I6 as light-brown solids. Synthesis of I7–I9 3-bromopropyl 2-bromoacetate (for I7 ), bis(3-bromopropyl) succinate (for I8 ), or 3-bromopropyl 4-bromobutanoate (for I9 ) (0.5 eq. ), 6-hydroxyindanone (0.70 g, 1 eq. ), N( n -C 4 H 9 ) 4 Br (0.1 eq. ), and K 2 CO 3 (2 eq.) in dry DMF (20 ml) were stirred at 65 °C overnight under N 2 . Upon cooling to RT, dry CH 2 Cl 2 (50 ml) was added, solids were filtered off and the filtrate was washed with H 2 O (3 × 100 ml). The organic fractions were dried over MgSO 4 , filtered and dried under reduced pressure to afford I7 – I9 as brown solids. McMurry coupling TiCl 4 (6 eq.) was added to a stirred suspension of Zn powder (12 eq.) in dry THF (~50 ml) over 10 min at 0 o C. The resulting slurry was refluxed for 1.5 h. To the refluxing mixture I4 , I5 , I6 , I7 , I8 or I9 (0.6 g, 1 eq.) in THF (~100 ml) was added over ~5 h by syringe pump. The reflux was continued for 20–40 min. The mixture was cooled to RT, poured into a saturated aqueous solution of NH 4 Cl and the product was extracted with CH 2 Cl 2 . The organic fractions were dried over MgSO 4 , and I10 – I15 were obtained as yellow solids after solvent removal. Reduction of esters I10–I15 to diols I16–I21 LiAlH 4 (2 eq.) was added to a stirred solution of I10 – I15 (0.4 g, 1 eq.) in dry THF (~40 ml) under N 2 . The resulting mixture was refluxed for 4 h. After cooling to RT, the reaction was quenched with H 2 O and the solids were filtered off. The filtrate was evaporated, dissolved in CH 2 Cl 2 , washed with H 2 O and dried over MgSO 4 . The product ( I16 – I21 ) obtained after CH 2 Cl 2 removal was used without purification. Bromination of diols I16–I21 to dibromides I22–I27 PPh 3 (4 eq.) was added carefully to a stirred solution of I16 – I21 (0.3 g, 1 eq.) and CBr 4 (4 eq.) in CH 2 Cl 2 (20 ml) containing five drops of acetone. The resulting mixture was stirred for 10–15 min and purified immediately by flash chromatography on silica with a gradient from hexanes to CH 2 Cl 2 . The product was further purified with preparative centrifugally accelerated radial thin-layer chromatography to afford pure I22 – I27 as yellow oils. Synthesis of Z1–Z6 Thiourea (4 eq.) and dibromides I22 – I27 (0.2 g, 1 eq.) in DMF (20 ml) were stirred at 80 °C under N 2 overnight. After cooling to RT, degassed 1 M NaOH aqueous solution (20 ml) was added under N 2 , the mixture was stirred at RT for 50 min, acidified with degassed 1 M HCl to pH=3 and the product was extracted with CH 2 Cl 2 . Drying with MgSO 4 , filtration and evaporation of CH 2 Cl 2 afforded dithiols I28 – I33 , which were oxidized immediately as follows. Solutions of I 2 and I28 – I33 in CHCl 3 were added simultaneously by syringe pump at the same rate over ~3 h to CHCl 3 (50 ml) containing N(C 2 H 5 ) 3 (1 ml). The mixture was poured in H 2 O, acidified to pH=3 with 1 M HCl, and unreacted I 2 was removed with Na 2 S 2 O 3 . The isolated organic fractions were dried over MgSO 4 . The crude product was purified with centrifugally accelerated radial thin-layer chromatography eluting with CH 2 Cl 2 /hexanes (2:3 mol) to afford pure Z 1 – Z 6 . Kinetic measurements The reduction kinetics was measured under pseudo-first-order conditions in phosphine (0.2–1 mM of PPh 2 CH 3 or 5 mM of PPh 3 and 20 μM for a disulphide) under rigorously anaerobic conditions. Because in acidic solutions, partial protonation of phosphine lowers its effective concentration, we measured the protonation constants of the phosphines, K p , in H 2 O:CH 3 CN (3:1 mol). We extracted K p from pseudo-first-order reduction rate constants of E 1 , E 2 and E 6 , k E pseudo , at different concentrations of triflic acid, (TfOH) ( Supplementary Table S7 ), by fitting them to equation (3) ([PR 3 ′] t is the total initial concentration of the phosphine and k E is the bimolecular rate constant for the phosphine reduction), assuming that the reduction is a single-barrier reaction. The validity of this assumption was confirmed by linearity of the [PR 3 ′] o / k E pseudo versus [H + ] plot ( Supplementary Figure S4 ), where [H + ] was calculated by equation (4). K p we measured for PPh 3 (480±40 M −1 ) is close to the literature value (~500 M −1 ) [49] ; K p for PPh 2 CH 3 has not been reported. Initial guesses for fitting measured k Z rate constants to equation (2) ( K s k 2 ′/ k −1 and k 2 / k −1 ), were obtained by linear least-squares fits (LSFs) of ( k E /2 k −1 ) −1 versus [H + ] (that is, by assuming k 1 Z = k E /2). The lsqnonlin function of Matlab was used to refine these guesses by non-linear LSFs to equation (2), which yielded more accurate values of k 1 Z than those underlying the initial guess of the fitting parameters. These new values were used to calculate ( k 1 Z / k −1 ) −1 and the new values of the fitting parameters K s k 2 ′/ k −1 and k 2 / k −1 from linear LSFs of ( k 1 Z / k −1 ) −1 versus [H + ] correlations (that is, similar to Fig. 3 ). The procedure was repeated until the relative change in k 1 Z between two sequential cycles of lsqnonlin fitting was <10 −5 . The uncertainty of k 1 Z was estimated from the Jacobian returned by lsqnonlin. [56] The uncertainties of K s k 2 ′/ k −1 and k 2 / k −1 were estimated from linear LSFs of the ( k 1 Z / k −1 ) −1 versus [H + ] data using the converged values of k 1 Z ( Supplementary Table S8 ). The reduction kinetics of 1 – 6 was measured on mixtures of different macrocycles, because there was no measureable effect on the reduction kinetics of any individual macrocycle from the presence of other macrocycles in the same reaction mixture. Based on the composition of the mixtures whose constituents could be conveniently separated ( Supplementary Table S3 ), either E -6,6′-bismethoxybiindanylidene or Z I10 ( Fig. 4 ) was used as an internal standard. They were chosen because of their availability in high purity, their chemical inertness towards all other components in the reaction mixtures and their retention times on reverse-phase HPLC. To prevent re-oxidation of the product dithiols by atmospheric oxygen HPLC-grade CH 3 CN and H 2 O used as reaction solvents were thoroughly sparged with N 2 before use. 1 H-NMR spectroscopy confirmed that CH 3 CN solutions of PPh 3 , and PPh 3 Me were stable for weeks when prepared under these conditions and stored in vials sealed under N 2 . Reactions were carried out in sealed vials, using a gas-tight syringe to withdraw ~100-μl aliquots for composition analysis by HPLC. These samples were transferred to clean vials and either analysed immediately or sealed under N 2 and stored at –35 °C until analysis. Reaction vials were held in a custom-made heating block with resistance heaters and a thermocouple connected to an active feedback temperature controller, which enabled the temperature of the reaction mixtures to be maintained with a stability of ±0.1 °C. The reaction temperature was recorded every 6 s. To prevent photoisomerization between E and Z isomers by ambient light, amber glass vials were used and all samples were kept away from light. No changes in E / Z ratios could be detected in samples stored for weeks under these conditions. Reaction mixtures were prepared by diluting combinations of stock solutions of the disulphides or their photostationary mixtures (for compositions of mixtures, see Supplementary Table S3 ) with CH 3 CN, water, aqueous TfOH, and phosphine in CH 3 CN to give a total absorbance of ~0.3, corresponding to ~20 μM total concentration of disulphide, a total volume of 800 or 1,200 μl, the desired concentrations of phosphine and TfOH, and a H 2 O/ CH 3 CN ratio of 3:1 (molar). Reaction mixtures were allowed to equilibrate to the temperature of the heating block before the addition of the phosphine solution. After the addition the reaction vial was shaken vigorously for ~2 s and returned to the thermostated heating block. Samples were then collected at regular intervals, as described above. Stock solutions of phosphines used were sufficiently concentrated so that the volume of the addition required was minimal (~10–20 μl out of the total 800–1,200 μl), minimizing cooling of the reaction mixture upon addition. DFT calculations of the reaction-path data in Fig. 1 All calculations were performed with Gaussian09.B01 and the 6-311+G(d) basis set; dissociation of the anthracene dimer (green) and methylethylidene cyclobutane (blue) were calculated with the uB3LYP functional in the gas phase; the remaining reactions utilized the B3LYP functional using SMD [53] as a continuum model of reaction solvent (H 2 O-parameterized SMD for ester and amide bond hydrolysis; methanol-parameterized SMD for degenerate methanolysis of O=P(OMe) 3 ). Ester and amid hydrolysis used five molecules of microsolvation, as described in Akbulatov et al . [48] The standard algorithm (Gaussian irc keyword) was used. Reaction-path calculations started from all conformers of the two transition states in both forward and reverse directions. Methylethylidene cyclobutane (blue) and the stationary points along its dissociation path have single conformer. For other reactions, transition states had more conformers than the reactant or the intermediate (that is, multiple conformers of the transition states lead to the same reactant or intermediate). In these cases, only the lowest-energy conformer was considered in ensemble averaging. Several conformers of the intermediate for ester and amide hydrolysis do not appear to be directly linked to either TS1 or TS2, and these conformers were excluded from ensemble averaging. IRC calculations toward the reactants or the products terminated 2–4 kcal/mol above the energy of separated reactants, or products, which is typical for bimolecular dissociation reactions. The value of the reaction coordinate corresponding to the reactants was determined by fitting the ~75% of the computed irc closest to the reactant end to a quadratic function and assigning to the reactants the value of the reaction coordinate corresponding to the minimum of this function. The intrinsic reaction coordinates (in units of bohr amu 0.5 ), which were unique for each irc, were rescaled to a uniform scale so that the reactants were assigned a value of -2; the TS1, -1; the intermediate 0 and the TS2, 1. The relationship between the intrinsic reaction-coordinate value and the uniform values was fitted to a quadratic equation to position the non-stationary points properly along the new uniform reaction path. On the new reaction-coordinate scale, the irc calculations terminated at the product side at values between 3 and 4.5 (the data plotted in Fig. 1a , main text, is truncated at 3). The electronic energies and the length of the internal coordinate ( q ) along the reaction path were fitted to a sixth-order polynomial with respect to the new uniform reaction-coordinate scale (because structures calculated along individual reaction path did not occur at the same values of the new reaction-coordinate scale). These functions were Boltzmann-averaged as described previously [48] and the results were fitted to a sixth-order polynomial to eliminate scatter, which arises because individual structures along reaction path had finite separation. This data is plotted in Fig. 1 . DFT calculations of externally constrained ensembles All calculations were performed with Gaussian09.B01 using Berny’s algorithm to locate stationary points. To ensure reliable compliances, very tight convergence criteria and ultrafine integration grids were used. Thermodynamic corrections to electronic energies of individual conformers were calculated statistical-mechanically in the harmonic oscillator/rigid rotor/ideal gas approximations. [57] Vibration frequencies <50 cm −1 were replaced with 50 cm −1 to avoid the artifactually large contribution of such modes to entropy. [57] Ensembles free energies were calculated as , where G min is the free energy of the conformational minimum, Δ G i is the free energy of conformer i relative to this minimum, and g i is its degeneracy. Energy barriers separating individual strain-free conformers were <4 kcal mol −1 (versus >20 kcal mol −1 for Δ G ‡o ), justifying calculations of ensemble properties and activation energies by Boltzmann statistics. The basis set superposition error (1.2 kcal/mol) was estimated as the difference of single-conformer electronic activation energy of the first step of the reduction of Et 2 S 2 by PPh 2 CH 3 calculated with 6-311+G(d) and B3LYP/6-311++G(3df, 2pd) basis sets in SMD [53] ( Supplementary Table S15 ). We calculated the activation free energy of the first step of PPh 3 and PPh 2 CH 3 reduction of Et 2 S 2 coupled to massless infinitely compliant constraining potential ( Fig. 7b ) by equation (5), [3] which is derived from the statistical-mechanical formulation of the transition state theory, [57] where E i , TC i and q i are the electronic energy, thermodynamic correction and the length of the constrained coordinate in conformer i and summation is overall conformational minima that exist in mechanical equilibrium with constraining force f (‡ signifies the transition state). [23] This formalism is applicable for constrained molecules in this study, because a molecule plus its constraint are stationary points and an infinitely compliant potential does not perturb the vibration frequencies of the coupled molecule. [3] At least two strategies exist to calculate the parameters of equation (5): First, direct computation of E i ( f ), TC i ( f ) and q i ( f ) by solving the system of equations , such that the solution satisfies the definition of the local minimum or the first order saddle point. Here Q is a vector of 3N-6 non-redundant internal coordinates of the molecule with Q (1) being the constrained molecular coordinate (note that the system of equations does not generally have a unique solution, that is, even a single conformer would have several geometries that would satisfy the system of equations). This strategy was used successfully [20] , [21] , [22] , [24] to calculate electronic energies of activation of cyclobutene ring-opening and analogous reactions in single ground and transition-state conformers of small molecules. This approach is particularly useful for MD simulations, but its current implementations remain too expensive for optimizations of thermodynamic states comprising dozens or hundreds of individual conformers. Alternatively, there is a two-step procedure based on the highly efficient relaxed potential energy scan (rPES) algorithm implemented in Gaussian. In this approach, the electronic energy and thermodynamic corrections are calculated for several values of the constrained distance, q , for example, E i ( q ), TC i ( q ). In Gaussian, the correlation between the length of the constrained coordinate and its restoring force, q i versus f i is obtained automatically, that is, rPES produces both E i ( q ) and E i ( f ) correlations. Depending on the size of the increment of q used in potential energy scans, the E i ( f ) and TC i ( f ) correlations may be sampled at different values of f for different conformers, for example, electronic energy and thermodynamic corrections for conformer 1 may be calculated at restoring forces of 10, 22, 35, 47, 60,…pN; whereas the same parameters for conformer 2 may be calculated at restoring forces of 12, 30, 50, 65,...pN. As an infinitely compliant potential can impose the same force on all conformers regardless of the length of their constrained distance, discrete values of E i ( f i ), TC i ( f i ) and q i ( f i ) thus obtained were interpolated using the spline algorithm to yield values of E i ( f ), TC i ( f ) and q i ( f ) at the same force for all conformers. For each conformer, the raw scan data (electronic energies, thermodynamic corrections, compliances, H 3 C … CH 3 ( q ) and two S … CH 2 ( q l ) separations) were interpolated to obtain uniform force increment of 1 pN using the interp1 function of Matlab 7.13.0.564. The interpolated data were fitted to a sixth-order polynomial to smooth it. Conformers of Et 2 S 2 and the corresponding transition states were searched systematically, as previously described. [25] Analytical frequency calculations yielded 0 (reactants) or 1 imaginary frequency (transition states) for all converged structures. Supplementary Tables S16–S18 list key parameters for the conformers. The calculated activation free energy of the first step of reduction of Et 2 S 2 with PPh 2 CH 3 and PPh 3 in H 2 O are 15.7 and 19.2 kcal/mol, respectively, versus 14.9 and 17.1 kcal/mol measured in 0.1 M NaOH in H 2 O/dioxane (3:1 mol). [49] , [50] , [51] We calculated the restoring forces of the local coordinate, f l in each conformer of Et 2 S 2 as f λ c l /λ l , [3] where λ l is (force-dependent) compliance of local coordinate l , and λ c l is the coupling coefficient [58] between this coordinate and the constrained distance. All compliances were derived from analytical Hessians computed at force f. Calculations with B3LYP/6-311+G(d) and B3LYP/6-311++G(3df, 2pd) basis sets resulted in nearly identical force-extension curves and the relationship between the stretching and local forces of the ensemble of Et 2 S 2 ( Supplementary Fig. S5 ). The force-induced barrier lowering results exclusively from the decrease in the potential energy of the constraining potential that accompanies the formation of the transition state ( Supplementary Fig. S2 ); the constraining potential destabilizes the transition state to a larger extent than the reactant, accounting for barrier-raising contribution of the molecular strain energy. Molecular compliances were calculated as BH −1 B T , where H is the Cartesian Hessians (obtained from frequency calculations on converged geometries), B is a truncated Wilson matrix (having three rows, for the constrained H 3 C … CH 3 and the two local coordinates, S … CH 2 , q l ), and −1 signifies inversion by the ‘back-slash’ numerical algorithm of Matlab. DFT calculations of the macrocycles Conformers of all Z and E macrocycles (reactants) were first searched by a Monte-Carlo algorithm with the MMFF force field in VeraChem. The conformers were then reoptimized at BLYP/6-31+G(d) with density autofitting in gas phase, and unique structures reoptimized at B3LYP/6311+G(d) in H 2 O-parameterized SMD, followed by wavefunction stability test and analytical frequency calculations. The transition state conformers were generated similarly but with the scissile S … S and forming S … P bonds frozen at 2.65 and 2.35 Å, respectively. The unique conformers were reoptimized at BLYP/6-31+G(d) with density autofitting. For the unique geometries, the constraints were removed, analytical frequencies were calculated to guide Berny’s search and the geometries were reoptimized at B3LYP/6-31+G(d) in H 2 O-parameterized SMD, followed by wavefunction stability test ( E isomers only) and analytical frequency calculations. Finally, conformers within 2.5 kcal/mol of the global conformational minimum of each state were reoptimized at B3LYP/6-311+G(d) in H 2 O-parameterized SMD. All transition-state conformers manifested a single imaginary frequency between −60 and −170 cm −1 . Supplementary Tables S13 and S14 list the key parameters of the reactant and transition states, and Supplementary Tables S15–S17 list the key parameters of individual conformers of the macrocycles. How to cite this article: Tian, Y. et al . Model studies of force-dependent kinetics of multi-barrier reactions. Nat. Commun. 4:2538 doi: 10.1038/ncomms3538 (2013).